A polymer tandem solar cell with 10.6% power conversion efficiency An effective way to improve polymer solar cell efficiency is to use a tandem structure, as a broader part of the spectrum of solar radiation is used and the thermalization loss of photon energy is minimized. In the past, the lack of high-performance low-bandgap polymers was the major limiting factor for achieving high-performance tandem solar cell. Here we report the development of a high-performance low bandgap polymer (bandgap <1.4 eV), poly[2,7-(5,5-bis-(3,7-dimethyloctyl)-5H-dithieno[3,2-b:2′,3′-d]pyran)-alt-4,7-(5,6-difluoro-2,1,3-benzothia diazole)] with a bandgap of 1.38 eV, high mobility, deep highest occupied molecular orbital. As a result, a single-junction device shows high external quantum efficiency of >60% and spectral response that extends to 900 nm, with a power conversion efficiency of 7.9%. The polymer enables a solution processed tandem solar cell with certified 10.6% power conversion efficiency under standard reporting conditions (25 °C, 1,000 Wm −2 , IEC 60904-3 global), which is the first certified polymer solar cell efficiency over 10%. Organic photovoltaics (OPV) is an emerging photovoltaics (PV) technology with promising properties such as low cost, flexibility, light weight, transparency and large-area manufacturing compatibility [1] , [2] , [3] , [4] , [5] , [6] . Polymer solar cells (PSCs) based on conjugated polymers as electron donor materials blended with [6,6]-phenyl-C 71 -butyric acid methyl ester (PC 71 BM) as an electron acceptor material have been the leading candidates in OPV in the past several years and achieved ~8% power conversion efficiency (PCE) using a single bulk heterojunction device structure [7] , [8] , [9] , [10] . To use solar radiation more effectively, a useful approach is to stack multiple photoactive layers with complementary absorption spectra in series to make a tandem PSC [11] , [12] , [13] , [14] , [15] , [16] , [17] , [18] , [19] . Typically, for a double-junction cell, such a tandem structure consists of a front cell with a high-bandgap material, an interconnecting layer, and a rear cell with a low-bandgap (LBG) material [11] , [12] , [13] , [14] , [15] , [16] , [17] , [18] , [19] . Compared with a single-junction device using low-bandgap materials, the multijunction/tandem structure can reduce thermalization loss of photonic energy during the photon-to-electron conversion process, and maximize the open circuit voltage ( V OC ). The high bandgap material in the front cell, which is responsible for the absorption of high-energy photons provide higher V OC than the low bandgap material. Therefore, by adopting polymers with matched absorption spectra, a tandem solar cell can effectively utilize the photonic energy and optimize open-circuit voltage, which leads to high PCE. In serial connected tandem solar cell, it is very obvious that subcell current balancing is critical for achieving high efficiency [18] . Inorganic multi-junction/tandem solar cells have gone a long way and the latest cell efficiency of 43.5% have been certified [20] , which shows the great potential of tandem solar cell. For polymer tandem solar cells, Hadipour et al. [13] demonstrated a polymer tandem solar cell consisting of two subcells with two different materials with about 0.57% efficiency in 2006, which is higher than each of the subcell’s efficiencies. In 2007, Kim et al. used a new interconnecting layer structure to bridge two higher performance single junction polymer PV cells to realize a tandem structure with 6.5% PCE [14] . More recently, Janssen et al. [18] has studied the effect of current matching on the tandem device performance, which provides more insight to achieve high-performance tandem PSC. However, the polymer tandem solar cells’ performance has been limited to around 7% efficiency in the last 4 years mainly due to the lack of high-performance low-bandgap polymers [15] , [16] , [17] , [18] with high V OC and high external quantum efficiency (EQE) at long wavelengths. Recently, we designed a new low bandgap polymer PBDTT-DPP with improved quantum efficiency (EQE~;50%) at long wavelength, and successfully achieved an inverted tandem PSC [17] with PCE of certified 8.6% ( [19] , [21] ). These progresses have translated the tandem polymer PV from a concept to a real OPV technology breakthrough, and paved a solid ground for achieving higher efficiencies in the future. With the progress in inter-connecting layer development, the main technical obstacle to break 10% barrier with a tandem PSC is the low bandgap polymer. The high bandgap cell in an inorganic multi-junction solar cell typically has a band gap of ~1.9 eV. In the PSC field, several polymers with ~1.9 eV such as poly-(3-hexylthiophene) (P3HT) [2] and poly N-9″-hepta-decanyl-2,7-carbazole-alt-5,5-(4′,7′-di-2-thienyl-2′,1′,3′-benzothiadiazole) [22] have shown excellent performance, with short circuit current density ( J SC ) over 10 mA cm −2 , and high EQE of ~70% from 400−600 nm. With 70% fill factor (FF) and over 1.5 V open circuit voltage in a tandem cell, a J SC of 10 mA cm −2 will lead to over 10% PCE. To achieve 10 mA cm −2 J SC in a low bandgap polymer cell between 600 nm and longer wavelength, an EQE close to 90% are required for polymer that absorbs up to 800 nm (~1.55 eV), or 60% for one that absorbs to 900 nm (~1.38 eV) [23] . So far, with a low bandgap cell of ~1.4 eV, the PSC shows only 5–6% PCE [19] , [24] , [25] , [26] , [27] . Particularly, most of the low bandgap polymers show low quantum efficiency (<50%) [19] , [21] and are not able to satisfy the requirement for a tandem cell. In this article, we report a low bandgap polymer design and the development of high performance single junction and double-junction PSCs. Starting from the reported LBG polymer poly[2,6-(4,4-bis-(2-ethylhexyl)-4H-cyclopenta[2,1-b;3,4-b′]-dithiophene)-alt-4,7-(2,1,3-benzothiadiazole)] (PCPDT-BT) [26] , [27] , [28] , we introduced two strong electron-withdrawing fluoroine atoms on the benzothiadiazole (BT) unit to form the difluorobenzothiadiazole (DFBT) unit to lower the highest occupied molecular orbital (HOMO) level [9] , [29] , [30] , [31] , [32] , [33] . The resulted polymer—poly[2,6-(4,4-bis-(2-ethylhexyl)-4H-cyclopenta[2,1-b;3,4-b′]-dithiophene)-alt-4,7-(2,1,3-difluorobenzothiadiazole) (PCPDT-DFBT) shows significantly enhanced V OC and photovoltaic performance. Second, we inserted a strong electron-donating oxygen atom into the cyclopentadithiophene (CPDT) unit to form the dithienopyran (DTP) unit to further lower the bandgap. These two strategies lead to a novel polymer poly[2,7-(5,5-bis-(3,7-dimethyl octyl)-5H-dithieno[3,2-b:2′,3′-d]pyran)-alt-4,7-(5,6-difluoro-2,1,3-benzothiadiazole)] (PDTP-DFBT) with a bandgap of 1.38 eV, which also shows a high hole mobility and deep HOMO level. Single-junction devices based on PDTP-DFBT show high quantum efficiency of >60% from 710 to 820 nm and the spectral response extends to 900 nm. This leads to a PCE of 7.9%. The polymer also enables over 10 mA cm −2 J SC in tandem solar cells. As a result, certified 10.6% PCE is achieved under standard reporting conditions (25 °C, 1,000 Wm −2 , IEC 60904-3 global). Polymers design and characterization The chemical structure of PCPDT-BT, PCPDT-DFBT and PDTP-DFBT are shown in Fig. 1a . The synthesis procedures can be found in the Methods and Supplementary Fig. S1 . All polymers showed molecular weight of around 20 kDa and poly dispersity index of around 2.5. The ultraviolet-visible absorption spectra of these polymers in solid state are shown in Fig. 1b . As shown in the figure 1b, the main absorption range of PCPDT-BT covers from 500 to 850 nm; the absorption onset is located at around 850 nm, indicating an optical bandgap of 1.48 eV. Interestingly, by adding two F atoms onto the BT unit, the absorption spectrum of the new polymer PCPDT-DFBT shows a blue shift of around 30 nm (bandgap of around 1.51 eV), whereas the addition of F atoms did not affect the absorption spectrum of other reported polymer systems [9] , [29] , [30] , [31] , [32] , [33] . To further lower the bandgap to match a P3HT-based wide bandgap cell in a tandem structure, a strong electron-donating oxygen atom is introduced into the CPDT unit to form the DTP unit. By co-polymerizing with the strong electron-withdrawing DFBT unit, the polymer PDTP-DFBT shows significantly lower bandgap. The absorption spectrum of PDTP-DFBT is ~80 nm red-shifted ( Fig. 1b ) compared with PCPDT-DFBT and the bandgap is calculated to be 1.38 eV. The HOMO and lowest unoccupied molecular orbital level (LUMO) energy levels of the three polymers were determined by cyclic voltammetry (CV), and the results are shown in Fig. 1c . The HOMO and LUMO levels of PCPDT-BT are located at −5.18 and −3.56 eV, respectively. After adding two F atoms, PCPDT-DFBT shows a much deeper HOMO level (−5.34 eV) whereas the LUMO level (−3.52 eV) is almost unchanged. The deeper HOMO level of PCPDT-DFBT is desired to enhance the V OC , the similar LUMO level satisfies the exciton dissociation requirement. After adding the O atom, PDTP-DFBT shows slightly higher HOMO level (−5.26 eV) and lower LUMO (−3.61 eV), agrees with the lower optical bandgap. All the measured CV results are in accordance with density functional theory (DFT) calculations ( Supplementary Fig. S2 ). It should be noted that the LUMO difference between polymer (~−3.6 eV) and PCBM (~−4.0 eV) [19] is about 0.4 eV, there are sufficient driving force to dissociate the exciton at the bulk heterojunction interface [3] . 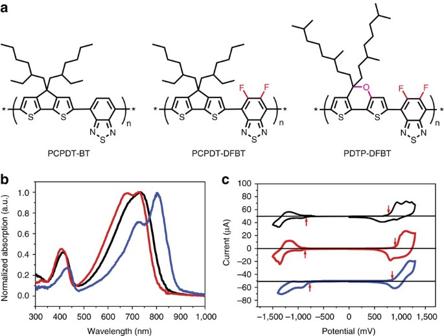Figure 1: Characterization of three DT-BT-based polymers. (a) Chemical structures of three different polymers (PCPDT-BT, PCPDT-DFBT and PDTP-DFBT) based on DT-BT backbone. (b) Normalized absorption spectra of the three polymers PCPDT-BT (black line), PCPDT-DFBT (red line) and PDTP-DFBT (blue line) spin-coated on glass substrate. (c) Electrochemical cyclic voltammogram of PCPDT-BT (black line) PCPDT-DFBT (red line) and PDTP-DFBT (blue line). The red arrows indicate the potential onset of the oxidation or reduction reactions in the electrochemical measurements. On the basis of equation (see Methods) it can be calculated the HOMO and the LUMO for PCPDT-BT are −5.18 and −3.56 eV, respectively; for PCPDT-DFBT, the HOMO and LUMO are −5.34 and −3.52 eV, respectively; for PDTP-DFBT, the HOMO and LUMO are −5.26 and −3.61 eV, respectively. a.u., arbitrary unit. Figure 1: Characterization of three DT-BT-based polymers. ( a ) Chemical structures of three different polymers (PCPDT-BT, PCPDT-DFBT and PDTP-DFBT) based on DT-BT backbone. ( b ) Normalized absorption spectra of the three polymers PCPDT-BT (black line), PCPDT-DFBT (red line) and PDTP-DFBT (blue line) spin-coated on glass substrate. ( c ) Electrochemical cyclic voltammogram of PCPDT-BT (black line) PCPDT-DFBT (red line) and PDTP-DFBT (blue line). The red arrows indicate the potential onset of the oxidation or reduction reactions in the electrochemical measurements. On the basis of equation (see Methods) it can be calculated the HOMO and the LUMO for PCPDT-BT are −5.18 and −3.56 eV, respectively; for PCPDT-DFBT, the HOMO and LUMO are −5.34 and −3.52 eV, respectively; for PDTP-DFBT, the HOMO and LUMO are −5.26 and −3.61 eV, respectively. a.u., arbitrary unit. Full size image Single junction solar cell devices Single junction photovoltaic cells based on the three polymers (and PC 71 BM as acceptor) were fabricated in an inverted device structure [34] , [35] , [36] , [37] , [38] . The PV performances are shown in Fig. 2a . For PCPDT-BT, the device showed a V OC of 0.62 eV and a J SC of 10 mA cm −2 , but the FF was only 50%. For PCPDT-DFBT, the V OC of the device was increased significantly to 0.85 V, as adding the F atoms lowered the HOMO level of the polymer ( Fig. 1c ). Both J SC and FF increased slightly compared with PCPDT-DFBT device. Upon the insertion of the electron-donating oxygen atom, the PDTP-DFBT-based devices showed significantly enhanced J SC of 17–18 mA cm −2 , which is among the highest reported J SC in PSCs so far. At the same time it gave a relatively high V OC close to 0.7 V, indicating the energy level tuning was successful to balance photocurrent generation and photovoltage. The performance of devices based on these three polymers is summarized in Table 1 . The EQE of these devices are shown in Fig. 2b . The EQE of PCPDT-BT and PCPDT-DFBT-based devices are around 40% peak (~35% average) and 50% peak (~45% average), respectively. The PDTP-DFBT-based devices showed much higher peak EQE over 60% (average ~55%), and the photoresponse extends to 900 nm. 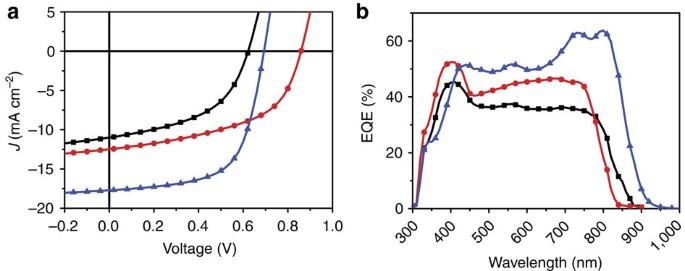Figure 2:J–Vcharacteristics and EQE of single-cell devices for three different polymers blending with PC71BM. (a)J–Vcharacteristics of single-cell devices PCPDT-BT:PC71BM (black line), PCPDT-DFBT:PC71BM (red line) and PDTP-DFBT:PC71BM (blue line) under simulated AM1.5G illumination from a calibrated solar simulator with irradiation intensity of 100 mW cm−2. (b) EQE of the corresponding devices, PCPDT-BT:PC71BM (black line), PCPDT-DFBT:PC71BM (red line) and PDTP-DFBT:PC71BM (blue line). Figure 2: J–V characteristics and EQE of single-cell devices for three different polymers blending with PC 71 BM. ( a ) J–V characteristics of single-cell devices PCPDT-BT:PC 71 BM (black line), PCPDT-DFBT:PC 71 BM (red line) and PDTP-DFBT:PC 71 BM (blue line) under simulated AM1.5G illumination from a calibrated solar simulator with irradiation intensity of 100 mW cm −2 . ( b ) EQE of the corresponding devices, PCPDT-BT:PC 71 BM (black line), PCPDT-DFBT:PC 71 BM (red line) and PDTP-DFBT:PC 71 BM (blue line). Full size image Table 1 Three different polymers’ parameters and their single junction devices performance when blending with PC 71 BM. Full size table Plasmon mapping based on energy-filtered transmission electron microscopy (EFTEM) was used to investigate the morphology of active layer [39] , [40] , [41] , [42] . The electron energy loss spectra of PDTP-DFBT and PDTP-DFBT:PC 71 BM are shown in Supplementary Fig. S3 . It can be seen that the polymer and blend system has a peak around 22.5 and 24.2 eV, respectively, which are consistent with the previous reports [39] , [40] , [41] , [42] , where the plasmon peak of [6,6]-phenyl-C 71 -butyric acid methyl ester (PC 71 BM) was found to be around 26 eV ( [39] , [40] , [41] , [42] ). Therefore, EFTEM enables us to use 20 and 30 eV energy loss to distinguish polymer and fullerene-rich domain, respectively, and provide more detailed morphology information than traditional TEM technique. The energy loss images of these three polymers blended with PC 71 BM at energy loss of 20 and 30 eV are shown in Fig. 3 . The energy loss images at 20 and 30 eV for PCPDT-BT: PC 71 BM and PCPDT-DFBT: PC 71 BM active layers (using chlorobenzene (CB) with 3% (vol.) 1, 8-diiodooctane (DIO)) are shown in Fig. 3b , respectively. Nanoscale fibril features were clearly seen from on both polymer blend films, indicating nice phase separation of polymer and fullerene for PCPDT-BT and PCPDT-DFBT system. On the other hand, it can be found that the PC 71 BM-rich domain (the dark region in 20 eV energy loss image, and bright region in 30 eV energy loss image) are as large as ~200 nm, which could be not good enough for charge separation and transport. The PDTP-DFBT: PC 71 BM film shows finely phase separation with the feature size of about 20–30 nm, and it is achieved using pure dichlorobenzene (DCB) solvent without the assistance of solvent additive ( Fig. 3h ). This type of morphology is expected to improve charge separation and transport [10] , [22] . For comparison, the zero loss images, formed with only elastically scattered electrons [39] , have also been collected. 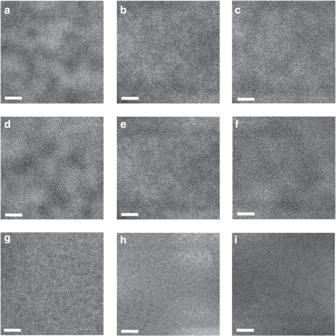Figure 3: The films’ morphology by energy-filtered TEM of polymer:fullerene blending films. (a–c) The energy loss image for PCPDT-BT:PC71BM spin-casted from CB solvent with DIO at energy loss of 0, 20 and 30 eV, respectively; (d–f) The energy loss image for PCPDT-DFBT:PC71BM spin-casted from CB solvent with DIO at energy loss of 0, 20 and 30 eV, respectively; (g–i) The energy loss image for PDTP-DFBT:PC71BM spin casted from DCB at energy loss of 0, 20 and 30 eV, respectively. The scale bars, 200 nm. Figure 3a,d and g are the zero loss images of PCPDT-BT:PC 71 BM, PCPDT-DFBT:PC 71 BM and PDTP-DFBT:PC 71 BM films, respectively. The zero loss images show the similar trend as plasmon energy loss mapping, with PBDT-DFBT:PC 71 BM owns a finer structure without large aggregation domain. Figure 3: The films’ morphology by energy-filtered TEM of polymer:fullerene blending films. ( a – c ) The energy loss image for PCPDT-BT:PC 71 BM spin-casted from CB solvent with DIO at energy loss of 0, 20 and 30 eV, respectively; ( d – f ) The energy loss image for PCPDT-DFBT:PC 71 BM spin-casted from CB solvent with DIO at energy loss of 0, 20 and 30 eV, respectively; ( g – i ) The energy loss image for PDTP-DFBT:PC 71 BM spin casted from DCB at energy loss of 0, 20 and 30 eV, respectively. The scale bars, 200 nm. Full size image Transport property is critically important for photovoltaic devices. Space-charge-limited current (SCLC) method was used to derive the hole mobilities of these three polymers. Hole-only devices were fabricated and the SCLC results are shown in Supplementary Fig. S3 . On the basis of equation 2 (see Methods) the mobilities are estimated to be 5.1 × 10 −4 , 4.8 × 10 −4 and 3.2 × 10 −3 cm 2 V −1 s −1 for PCPDT-BT, PCPDT-DFBT and PDTP-DFBT, respectively. The carrier mobilities in the polymer, however, could be affected by morphology, field, recombination or carrier densities effect in polymer:fullerene bulk heterojunction active layers under operating conditions. To get reliable charge carrier mobility of the blending system, photo-induced charge carrier extraction in a linearly increasing voltages (Photo-CELIV) measurements have been conducted in bulk heterojunction solar cells based on the three systems [43] , [44] . The maximum voltage is 2 V in our experiment, with active layer thickness ~100 nm, the maximum electric field is thus ~2 × 10 5 V cm −1 . And the charge carriers were extracted after 3 μs fixed delay time. The Photo-CELIV results are shown in Fig. 4 , where the t max (the time when the extraction current reaches its maximum value) for PCPDT-BT:PC 71 BM, PCPDT-DFBT:PC 71 BM and PDTP-BT:PC 71 BM are 7.1, 2.8 and 1.1 μs, respectively. 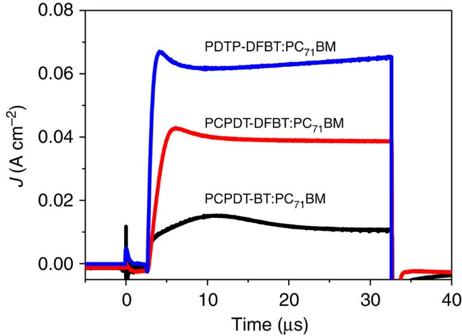Figure 4: Photo-CELIV of solar cells with different polymers blending with PC71BM. The delay times are 3 μs. And thetmax(the time when the extraction current reaches its maximum value) for PCPDT-BT:PC71BM, PCPDT-DFBT:PC71BM and PDTP-BT:PC71BM are 7.1, 2.8 and 1.1 μs, respectively. The device structure is ITO/ZnO/Polymer:PC71BM/MoO3/Ag. Figure 4: Photo-CELIV of solar cells with different polymers blending with PC 71 BM. The delay times are 3 μs. And the t max (the time when the extraction current reaches its maximum value) for PCPDT-BT:PC 71 BM, PCPDT-DFBT:PC 71 BM and PDTP-BT:PC 71 BM are 7.1, 2.8 and 1.1 μs, respectively. The device structure is ITO/ZnO/Polymer:PC 71 BM/MoO 3 /Ag. Full size image The charge mobility can then be calculated to be 1.2 × 10 −5 , 7.4 × 10 −5 and 6.7 × 10 −4 cm 2 V −1 s −1 for PCPDT-BT:PC 71 BM, PCPDT-DFBT:PC 71 BM and PDTP-BT:PC 71 BM, respectively (equation 3, see Methods). The qualitative charge carrier mobility data in the blend systems thus show the same trend, but are lower than those in pure polymer cases, which is consistent with the larger disorder in bulk heterojunction film. The PDTP-BT:PC 71 BM owns a higher charge carrier mobility than the other two polymer systems, which could contribute to the higher PV performance. For more details of SCLC and Photo-CELIV, please see Methods . Tandem devices based on P3HT:ICBA and PDTP-DFBT:PCBM From the analysis of spectral coverage and the single junction solar cell result, PDTP-DFBT shows high potential for application in tandem solar cells as a rear cell the tandem structure is shown in Fig. 6a. In a tandem structure, a high bandgap polymer, P3HT, combined with Indene-C 60 Bisadduct (ICBA) fullerene are selected as front cell active materials, and the low bandgap polymer PDTP-DFBT with PC 61 BM or PC 71 BM are selected as the rear cell active materials. Sol-gel processed ZnO is used as the electron transport layer, and PEDOT:PSS and MoO 3 are used as the hole transport layer for the front and rear cells, respectively. The inverted tandem structure was chosen because of its advantages of a simple, robust device fabrication process and better stability [8] , [34] , [35] , [36] , [37] . 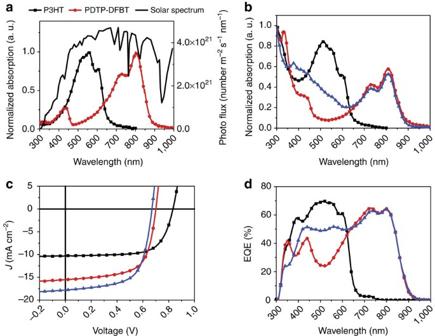Figure 5: Absorption and device performance. (a) Absorption spectra of P3HT and PDTP-DFBT and solar spectrum. (b) Absorption spectra of P3HT:ICBA (black line), PDTP-DFBT:PC61BM (red line), PDTP-DFBT:PC71BM (blue line) blend. (c)J–Vcurve of P3HT:ICBA (black line), PDTP-DFBT:PC61BM (red line), PDTP-DFBT:PC71BM (blue line) under AM1.5G illumination from a calibrated solar simulator with an irradiation intensity of 100 mWcm2(one Sun). (d) EQE of P3HT:ICBA (black line), PDTP-DFBT:PC61BM (red line), PDTP-DFBT:PC71BM (blue line)-based single cell devices. Figure 5a shows the ultraviolet-visible absorption spectra of P3HT and PDTP-DFBT in the solid state, and the solar radiation spectrum. It can be seen that these two polymers complementarily cover the solar spectrum from 350 to 900 nm with very little spectral overlap, which provides a favourable system combination for optimizing tandem cell performance through independent tuning of two subcells. IC 60 BA has been shown to be a successful acceptor for the high bandgap polymer P3HT [45] , [46] used in both single junction and tandem PSCs [19] . Two types of widely used fullerenes (PC 61 BM and PC 71 BM) with different absorption coefficients were examined [47] here to blend with the low bandgap polymer. The absorptions of polymers blended with acceptors are shown in Fig. 5b . When the low bandgap polymer PDTP-DFBT is blended with PC 61 BM, the absorption is enhanced slightly in the region of 300–400 nm due to the absorption of PC 61 BM, and the two subcells show little overlap. Whereas the PDTP-DFBT:PC 71 BM blend showed strong absorption in the entire visible region, and the overlap of two subcells is more significant. These different overlaps will affect the current match of the tandem solar cell, and thus the efficiency. Figure 5c shows the current versus voltage ( J–V ) characteristics of single-junction devices under AM1.5G illumination from a calibrated solar simulator with irradiation intensity of 100 mW cm −2 . All the single junction cells (P3HT:IC 60 BA, PDTP-DFBT:PC 61 BM, and PDTP-DFBT:PC 71 BM) show excellent performance. Specifically, the P3HT:IC 60 BA cell shows 6.1% PCE, and the PDTP-DFBT-based single junction cells show 7.1% and 7.9% PCE when blended with PC 61 BM and PC 71 BM, respectively. The difference comes from the J SC , which is mainly due to the different absorption coefficients of PC 61 BM and PC 71 BM in the region of 300–600 nm. The detailed parameters of the single cell are summarized in Table 2 . The EQE of P3HT:IC 60 BA, PDTP-DFBT:PC 61 BM, PDTP-DFBT:PC 71 BM are shown in the Fig. 5d . The wide bandgap polymer cell (P3HT:IC 60 BA) showed high quantum efficiency from 300–700 nm, with maximum EQE of 70% at about 520 nm. In both of the PDTP-DFBT-based single cells, the maximum EQE is 62% at ~800 nm, and EQE is over 60% from 710 to 820 nm. Figure 5: Absorption and device performance. ( a ) Absorption spectra of P3HT and PDTP-DFBT and solar spectrum. ( b ) Absorption spectra of P3HT:ICBA (black line), PDTP-DFBT:PC 61 BM (red line), PDTP-DFBT:PC 71 BM (blue line) blend. ( c ) J–V curve of P3HT:ICBA (black line), PDTP-DFBT:PC 61 BM (red line), PDTP-DFBT:PC 71 BM (blue line) under AM1.5G illumination from a calibrated solar simulator with an irradiation intensity of 100 mWcm 2 (one Sun). ( d ) EQE of P3HT:ICBA (black line), PDTP-DFBT:PC 61 BM (red line), PDTP-DFBT:PC 71 BM (blue line)-based single cell devices. Full size image Table 2 P3HT and PDTP-DFBT single junction cell and tandem solar cell performance. Full size table Accurate tandem cell measurement is a quite complicated procedure and extra care was taken to get reliable data [48] , [49] , [50] . EQE results were first measured in University of California, Los Angeles (UCLA) [48] , and the tandem devices were then measured using the One-Sun Multi-Source Simulator (recently established at National Renewable Energy Laboratory, (NREL)) based on UCLA EQE data [19] . The spectral mismatches associated with the re-measured EQEs and the simulator spectra were then recalculated. The spectral mismatches were found to be <0.2% different from those derived from the EQEs. The device structure, J–V , and EQE curves of the tandem solar cells are shown in Fig. 6 . To fine tune the balance of short-circuit current, acceptor materials with different absorption in the visible region (PC 61 BM versus PC 71 BM) were used for the low bandgap subcell. For simplicity, the corresponding devices are called Tandem 1 (PC 61 BM) and Tandem 2 (PC 71 BM), respectively. For the device Tandem 1, it shows a V OC of 1.53 V, J SC of 10.1 mA cm −2 , FF of 68.5%, and the PCE is 10.6%. The original I–V characteristic of the tandem 1 device as measured by NREL is shown in Fig. 7 . The EQE curves of the front and rare cells measured at NREL are shown in Supplementary Fig. S5 . For the device Tandem 2, the device shows a slightly lower V OC of 1.51 V, J SC of 9.80 mA cm −2 , FF of 69.2% and 10.2% PCE. The V OC ’s of the tandem cells are almost equal to the sum of single junction cells’ V OC , indicating the effectiveness of the interconnection layer. For example, the V OC for the front (P3HT:ICBA) and rear cell (PDTP-DFBT:PC 61 BM) are 0.84 and 0.70 V, respectively. The V OC of the tandem solar cell is 1.53 V, which is 0.01 V less than that of the front and rear cell V OC combination. The difference may come from (a) the small reisistance of the interconnecting layer, and/or (b) the slight V OC drop of the rear cell as the light intensity on the rear cell in the tandem configuration is weaker compared with one sun illumination. Therefore, the V OC of the tandem solar cell are almost equal to the sum of the single junction cells’ V OC , indicating the effectiveness of the interconnection layer. The slightly lower V OC in Tandem 2 with PC 71 BM also agrees well with the single junction device data. The EQEs of the devices Tandem 1 and 2 are shown in Fig. 6c . Using a different acceptor for the rear cell of the tandem solar cell, the EQE of both cells can be tuned. For the rear cell using PC 61 BM, the front P3HT cell shows the higher EQE and a J SC of 9.8 mA cm −2 derived from EQE. The rear cell shows lower EQE in the visible region, with well-matched integrated J SC of 9.8 mA cm −2 too. For the device Tandem 2, as PC 71 BM has strong absorption in the visible region, the photons not being absorbed after passing the front cell will be absorbed by the rear cell. Therefore, less photons (bounced back from the metal electrode) will be absorbed by the front cell. Accordingly, the EQE between 300 and 600 nm of the front cell will be reduced and the rear cell EQE will be increased. In the current case, after replacing the PC 61 BM with PC 71 BM in the rear cell, the maximum EQE of front cell is reduced from 70 to 65%. Finally, the integrated short-circuit current of the front cell is 9.5 mA cm −2 , whereas the integrated short-circuit current of the rear cell is 10 mA cm −2 . Tandem solar cells’ current is usually determined by the subcell with the lowest J SC ( [11] , [18] ). Therefore, although the device Tandem 2 shows excellent FF of 69.2% and V OC of 1.51 V, it shows a lower measured J SC of 9.8 mA cm −2 and gives a PCE of 10.2%. It is clear that choosing different fullerene derivatives to adjust current matching provides an effective tool to tune the performance of tandem PSCs. For each type of devices, we have tested about 100 devices, for the Tandem 1 (P3HT:ICBA/PDTP-DFBT:PC 61 BM), the highest is 10.6%, and the average PCE is 10.4%; for Tandem 2 (P3HT:ICBA/PDTP-DFBT:PC 71 BM), the highest PCE is 10.2%, and the average is 9.9%. These results show our devices have excellent reproducibility. In the present work, the PC 61 BM allows better decoupling of the two cells, which could make the tandem solar cell optimization easier. The successful application of PC 61 BM to achieve high-performance tandem cells also has the benefit of reducing the materials cost of PSCs [47] . 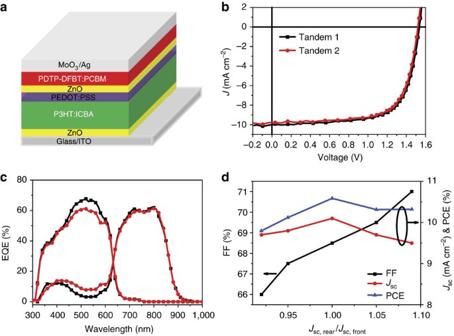Figure 6: Tandem devices structure and performance. (a) Device structure of the tandem solar cell (Glass/ITO/ZnO/P3HT:ICBA/PEDOT:PSS/ZnO/PDTP-DFBT:PCBM/MoO3/Ag). (b)J–Vcurve of P3HT:ICBA/PDTP-DFBT:PC61BM combination (Tandem 1) and P3HT:ICBA/PDTP-DFBT:PC71BM combination (Tandem 2) under AM1.5G illumination from a calibrated solar simulator with an irradiation intensity of 100 mWcm2(one Sun). (c) EQE of the tandem 1(black line) and 2 (red line) devices. A 700 and 550 nm light bias are used to get front and rear cell EQE, respectively. (d) The relationship of tandem cell FF and short circuit current (JSC) versus rear and front cell current ratio (JSC, rear/JSC,front). Figure 6: Tandem devices structure and performance. ( a ) Device structure of the tandem solar cell (Glass/ITO/ZnO/P3HT:ICBA/PEDOT:PSS/ZnO/PDTP-DFBT:PCBM/MoO 3 /Ag). ( b ) J–V curve of P3HT:ICBA/PDTP-DFBT:PC 61 BM combination (Tandem 1) and P3HT:ICBA/PDTP-DFBT:PC 71 BM combination (Tandem 2) under AM1.5G illumination from a calibrated solar simulator with an irradiation intensity of 100 mWcm 2 (one Sun). ( c ) EQE of the tandem 1(black line) and 2 (red line) devices. A 700 and 550 nm light bias are used to get front and rear cell EQE, respectively. ( d ) The relationship of tandem cell FF and short circuit current ( J SC ) versus rear and front cell current ratio ( J SC, rear / J SC,front ). 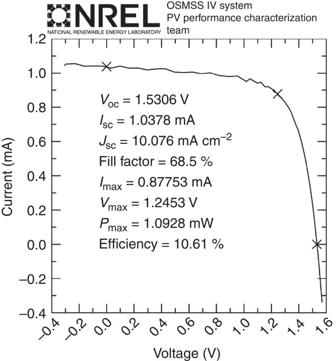Figure 7: OriginalI–Vcharacteristics of the Tandem 1 device. Device characteristics as measured by NREL. Full size image Figure 7: Original I–V characteristics of the Tandem 1 device. Device characteristics as measured by NREL. Full size image To systematically study the current match effect on the performance of the tandem solar cells, the thickness of the active layer and the choice of fullerene has been changed to tune the J SC of front and rear cells, the FF and the front and rear cell J SC ratio ( J SC, rear / J SC , front ) are shown in Fig. 6d ( V OC does not change with the active layer thickness and acceptor). The J SC ’s are derived from EQE measurements, and the ratios range from 0.92 to 1.10. It is clear that the J SC of the tandem solar cells follows the subcell with the limiting J SC as expected. The FFs of the tandem cell lie between the lower subcell FF (66%, rear) and the higher subcell FF (71%, front), and turn to follow that of the current limiting subcell. In our system, when the front and rear subcell J SC matches, the tandem devices showed the optimized performance ( Fig. 6d ) [49] , [50] . The J–V characteristics of the optimized tandem cell have been measured under different incident light intensities from 1.2 to 100 mW cm −2 (0.012–1 sun) using neutral density filters, and the results are shown in Fig. 8a . With no ultraviolet activation, even under low light, the fresh tandem solar cell shows high fill factor. In Fig. 8b , the J SC of the tandem cell is plotted as a function of incident light intensity. It is clear that the J SC is proportional to illuminated light intensity, indicating no substantial space charge build-up in the tandem device in both the two subcells and in the interconnecting layer [14] . The V OC and FF dependence on light intensity are shown in Fig. 8c , respectively. The FF of the tandem devices increased to 75% under low light intensity. This can be explained by the fact that under low intensity of light irradiation the recombination in the active layer is lower. The light intensity dependence of J SC , V OC and FF are very similar to that in reported high-performance single junction organic solar cell systems. Clearly, this will be the case when the two subcells each perform well, and are connected by an effective interconnecting layer. The maximum PCE reaches 11.1% at light intensity of 2.6 mW cm −2 (~0.02 sun). In addition, the tandem devices show relatively high stability. Supplementary Figure S6 indicates the devices performance degraded about 5% after 57 days. It is worth to mention that we observed some fluctuation in the NREL-measured tandem device J–V curve, but the fluctuations are at the 1% level or less, that is, within the requirements of a Class A simulator ( Supplementary Fig. S7 ). 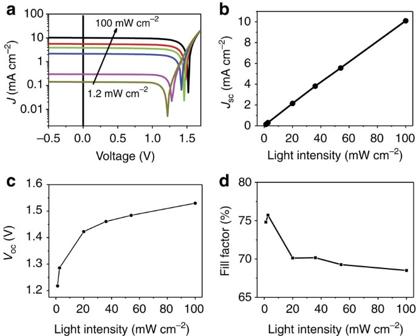Figure 8: Tandem solar cell performance parameters under low light intensity. (a)J–Vcurve of the tandem devices under different light intensity from 1.2 to 100 mW cm−2(0.012–1 Sun); (b–d) Variation of short circuit current (JSC), open circuit voltage (VOC), FF of the Tandem 1 device under different light intensity from 1.2 to 100 mW cm−2. Figure 8: Tandem solar cell performance parameters under low light intensity. ( a ) J–V curve of the tandem devices under different light intensity from 1.2 to 100 mW cm −2 (0.012–1 Sun); ( b – d ) Variation of short circuit current ( J SC ), open circuit voltage ( V OC ), FF of the Tandem 1 device under different light intensity from 1.2 to 100 mW cm −2 . Full size image In summary, we have demonstrated a solution processed tandem PSC with 10.6% PCE under standard reporting conditions (25 °C, 1,000 Wm −2 , IEC 60904-3 global). The devices consist of high-performance P3HT:ICBA front cell and PDTP-DFBT:PCBM rear cell. Looking into the future, as EQE at the 80% level has been demonstrated in single junction OPV cells, we believe this should be achievable in tandem OPV cells too. This ~30% enhancement will enable PSCs with ~14% PCE. Interfacial and active layer materials (including morphology control) will definitely have a critical role for achieving higher EQE. New donor and acceptor materials are needed to further improve V OC and J SC in tandem PSCs. The combination of these research approaches will ultimately drive the PSC efficiency to 15% and beyond in the near future. During the preparation of this manuscript, Heliatek in Germany demonstrated a 10.7% efficiency vacuum-processed small molecule organic tandem solar cell with an active area of >1 cm 2 ( http://www.heliatek.com/ ), both clearly show the importance of tandem structure in organic solar cells. Materials P3HT was purchased from Rieke Metals. PC 61 BM and PC 71 BM were purchased from Nano-C. The synthesis procedure of CPDT, DTP and DFBT units can be found in Zhu et al. [51] and Yoshimura and Ohya [52] . The polymers were synthesized as follow (see Supplementary Fig. S1 for the chemical reaction equations): PCPDT-DFBT: CPDT (0.337 g, 0.463 mmol) and DFBT (0.148 g, 0.449 mmol) were dissolved into 10 ml toluene in a flask protected by argon. The solution was flushed by argon for 10 min, then 8 mg of Pd 2 (dba) 3 and 16 mg of P(o-tol) 3 was added into the flask. The solution was flushed by argon again for 20 min. The oil bath was heated to 110 °C gradually, and the reaction mixture was stirred for 10 h at 110 °C under argon atmosphere. Then, the mixture was cooled down to room temperature and the polymer was precipitated by addition of 100 ml methanol and the precipitated solid was collected and purified by Soxhlet extraction (acetone for 24 h and then hexane for 24 h). The solid was then dissolved in 30 ml toluene and purified by chromatography on silica gel. Then the solution was concentrated to 10 ml and precipitated in methanol. The title polymer was obtained as dark purple solid, yield ~50%. The polymer can be readily dissolved into CB, DCB and so on. PCPDT-BT and PDTP-DFBT were synthesized using the same procedure. Electrochemical CV The electrochemical CV was conducted with Pt disk, Pt plate and Ag/AgCl electrode as working electrode, counter electrode and reference electrode, respectively, in a 0.1 mol l −1 tetrabutylammonium hexafluorophosphate (Bu 4 NPF 6 ) acetonitrile solution [1] . The polymer films for electrochemical measurements were coated from a polymer chloroform solution of concentration ~5 mg ml −1 . For calibration, the redox potential of ferrocene/ferrocenium (Fc/Fc + ) was measured under the same conditions, and it is located at 0.42 V to the Ag/AgCl electrode. It is assumed that the redox potential of Fc/Fc + has an absolute energy level of −4.80 eV to vacuum. The energy levels of the highest occupied (HOMO) and lowest unoccupied molecular orbital (LUMO) were then calculated according to the following equations: where E ox is the onset oxidation potential versus Ag/AgCl and E red is the onset reduction potential versus Ag/AgCl. Simulated results for the molecular orbital DFT calculations were executed to determine the electronic structures of the two polymers. Two repeating units of the polymers were used as the model compound in the simulation, and methyl groups were used instead of the long side chain. DFT calculations were done using HSE06/6-31G(d). The calculated HOMO/LUMO and bandgap for CPDT-BT, CPDT-DFBT and DTP-DFBT were −4.632/−2.714 and 1.918 eV, −4.827/−2.865 and 1.962 eV, −4.824/−2.914 and 1.910 eV, respectively. These results indicate that by adding two F atoms on the BT unit, CPDT-DFBT shows lower HOMO/LUMO levels and a larger bandgap than CPDT-BT due to the strong electron-withdrawing property of F atom; after further adding an O atom, DTP-DFBT shows lower HOMO/LUMO levels and a smaller bandgap than CPDT-BT. The simulation results are in accordance with experimental results. Morphology characterization EFTEM was used to characterize the morphology of the polymer:fullerene system. Thin films were analysed in a Titan Krios TEM equipped with an energy filter. By electron energy loss spectroscopy, plasmon energies of 20 and 30 eV were used to distinguish the polymer and PCBM, respectively. A slit width of 8 eV was used during the measurement. Mobilities measurement SCLC model measurement: Hole mobility was measured using the SCLC, using a diode configuration of ITO/PEDOT:PSS/polymer:/Au by taking current–voltage current in the range of 0–8 V and fitting the results to a space–charge-limited form, where the SCLC is described by where ε 0 is the permittivity of free space, ε r is the dielectric constant of the polymer, μ is the hole mobility, V is the voltage drop across the device and L is the polymer thickness. The dielectric constant ε r is assumed to be 3, which is a typical value for conjugated polymers. The thickness of the polymer films is measured by using a Dektek profilometer. The thickness of the polymer is ~100, 90 and 100 nm for PCPDT-BT, PCPDT-DFBT and PDTP-DFBT, respectively. The mobilities of these three polymers are 5.1 × 10 −4 , 4.8 × 10 −4 and 3.2 × 10 −3 cm 2 V −1 s −1 . Photo-induced charge carrier extraction in a linearly increasing voltages (Photo-CELIV) measurement: To further measure the mobility of the polymer:fullerene blend system, photo-induced charge carrier extraction in a linearly increasing voltages (Photo-CELIV) measurement was used to determine the charge carrier mobility in bulk heterojunction solar cells [44] . The device structure is ITO/ZnO/Polymer:PC 71 BM/MoO 3 /Ag. A 590-nm dye (Rhodamine Chloride 590) laser pumped by a nitrogen laser (LSI VSL-337ND-S) was used as the excitation source, the pulse energy and pulse width being about 3 μJ cm −2 and 4 ns, respectively. The current of the photodiode was first amplified by using a current amplifier (Femto DHPCA-100), then a preamplifier (SR SSR445A) and finally recorded using a digital oscilloscope (Tektronix DPO 4104). The t max values for PCPDT-BT:PC 71 BM, PCPDT-DFBT:PC 71 BM and PDTP-BT:PC 71 BM are measured to be 7.1, 2.8 and 1.1 μs, respectively. From the active thicknesses of 100, 90 and 100 nm, respectively, the mobilities of PCPDT-BT:PC 71 BM, PCPDT-DFBT:PC 71 BM and PDTP-BT:PC 71 BM are calculated to be 1.2 × 10 −5 , 7.4 × 10 −5 and 6.7 × 10 −4 cm 2 V −1 s −1 , respectively, based on the following equation [44] . where μ is the mobility, d is the thickness of the active layer, t max is the time when the extraction current is reached, A is the voltage rise speed A =d U /d t . In this measurement, the applied maximum voltage is 2 V, and U offset is chosen to be near the corresponding open-circuit voltage, the time t for voltage increase from U offset to maximum voltage is 30 μs, and j (0) is the capacitive displacement current [44] . Single-junction devices based on three different polymers The precleaned ITO substrates were first treated with ultraviolet-ozone for 15 min. ZnO nanoparticles were spin-coated on the ITO substrates. The synthesis process of ZnO nanoparticles can be found in You et al. , [53] Sun and Sirringhaus [54] and Beek et al. [55] Then the active layer was spin-coated on the ZnO surface; PCPDT-BT:PCBM (1:2), PCPDT-DFBT (1:2) and PDTP-DFBT:PCBM (1:2) were dissolved in CB or DCB with a concentration ranging from 5 to 10 mg ml −1 and with stirring at about 80 °C for at least 2 h before spin coating the active layer (heating is helpful to improve the solubility); for the PCPDT-BT and PCPDT-DFBT-based device, to improve the active layer morphology, 3% by volume DIO was added. After spin coating the active layer, the samples were transferred into the evaporation chamber for fabricating the MoO 3 /Ag electrode. Tandem devices fabrication The precleaned ITO substrates were first treated with ultraviolet-ozone for 15 min. The P3HT:IC 60 BA (1:1 weight ratio) in DCB solutions with various solid content were spin-casted at 800 r.p.m. for 30 s on top of a ~30 nm layer of ZnO [53] , [54] , [55] . The P3HT:ICBA film is formed through a slow growth process and the thickness is between 180 and 240 nm [2] . PEDOT:PSS layer was applied on the first subcell active layer and annealed at 150 °C for 10 min. Then a thin layer of ZnO film was spin-casted, followed again by thermal annealing at 150 °C for 10 min. The second subcell active layer of PDTP-DFBT:PCBM (PC 61 BM or PC 71 BM) (1:2) from an DCB solution was then spin-casted at 1,500 r.p.m. on top of the ZnO layer, the thickness of PDTP-DFBT is about 80–120 nm. To control the thickness to tune the short circuit current of front and rear cell, we varied the concentration of P3HT (18–22 mg ml −1 ) and PDTP-DFBT (5–7 mg ml −1 ) in the solution. The optimized thickness of the front and rear cell are about 220 and 100 nm, respectively. The inverted tandem PSC devices fabrication were completed by thermal evaporation of MoO 3 /Ag as the anode under vacuum at a base pressure of 2 × 10 –6 Torr. Tandem device characterization The device areas were measured in the NREL facility first using optical microscope, and the results range from 0.0998 to 0.104 cm 2 . EQEs were measured at UCLA and NREL, respectively. A 550- and 700-nm light bias was selected to excite the front and rear cells to measure the EQE of the rear and front cell, respectively. I–V measurements for the tandem cells were performed on the One-Sun Multi-Source Simulator of NREL first by using UCLA EQE data for spectral mismatch correction. The spectral mismatches associated with the re-measured EQEs and the simulator spectra were recalculated. In each case, the spectral mismatches were <0.2% different from those derived from the EQEs. Measurements in NREL were done at 1,000, 500 and 250 W m −2 with and without the mask (~0.04 cm 2 ) on a representative device. The J SC with the mask was about 2% lower than without the mask. Some of this difference is likely due to the extended source of the One-Sun Multi-Source Simulator light (as opposed to a point-like source) and the thickness of the mask relative to the size or the opening. For the different light intensity response measurement, neutral density filters were used to tune the light intensity, and a Si-diode was used to calibrate the light intensity. In examining the NREL certified J-V data, we observed some fluctuation in the J-V curve. We would like to explain the phenomenon as the following: 1) We believe part of the reason for the noise in the data is that there are multiple light sources (we have 9 separated light sources to control the spectrum) each with different intensity versus time characteristics. 2) Smooth I-V curves do not mean they are more accurate then IV curves with fluctuations. For example a halogen light source will give very smooth curves but the spectrum is a terrible match to the reference solar spectrum. 3) More importantly than the noise in the I-V curve was the fact that the spectrum was adjusted so that each cell was within 1% of its target photocurrent under the reference spectrum. 4) Furthermore, from the expansion data in Figure 7 (NREL data, see Figure S7), we can see the fluctuations are at the 1% level or less within the requirements of a Class A simulator. How to cite this article: You, J. et al. A polymer tandem solar cell with 10.6% power conversion efficiency. Nat. Commun. 4:1446 doi: 10.1038/ncomms2411 (2013).